Evidence for a weakening relationship between interannual temperature variability and northern vegetation activity Satellite-derived Normalized Difference Vegetation Index (NDVI), a proxy of vegetation productivity, is known to be correlated with temperature in northern ecosystems. This relationship, however, may change over time following alternations in other environmental factors. Here we show that above 30°N, the strength of the relationship between the interannual variability of growing season NDVI and temperature (partial correlation coefficient R NDVI-GT ) declined substantially between 1982 and 2011. This decrease in R NDVI-GT is mainly observed in temperate and arctic ecosystems, and is also partly reproduced by process-based ecosystem model results. In the temperate ecosystem, the decrease in R NDVI-GT coincides with an increase in drought. In the arctic ecosystem, it may be related to a nonlinear response of photosynthesis to temperature, increase of hot extreme days and shrub expansion over grass-dominated tundra. Our results caution the use of results from interannual time scales to constrain the decadal response of plants to ongoing warming. Previous research has documented a tight positive relationship between space-borne measurements of the Normalized Difference Vegetation Index (NDVI) by National Oceanic and Atmospheric Administration satellites and growing season temperature in the Northern Hemisphere (NH) [1] , [2] , [3] . This observation can be interpreted as an increase in photosynthesis in response to warmer climate conditions, and the observed ‘northern greening’ over the past 30 years has been extrapolated as a sign that northern ecosystems will continue to grow more and thus accumulate more carbon in a warmer world [4] , [5] . However, although future NH warming is projected to increase in the future [6] , the response of vegetation remains uncertain, as the relationship between temperature and vegetation productivity may change over time, given other environmental limitations [7] , [8] . Although direct warming is the most frequently discussed change in recent times, major changes to other climate attributes have been experienced by the northern vegetation over the last three decades [6] . The Palmer Drought Severity Index (PDSI), which is defined from a water-balance model forced with climate data, shows a significant increase in drought over the NH in the last several decades, and particularly in southern Europe and eastern Asia and Siberia [9] . Increased drought stress can modify the response of plant growth to temperature change [7] and was hypothesized to be a potential cause for the declined temperature sensitivity of tree growth in tree rings time series during the last part of the twentieth century [10] . The effect of climate drought on the temperature sensitivity of vegetation growth, however, may be partly alleviated by CO 2 -induced increase in vegetation water use efficiency [11] , [12] . In addition, some species can also gradually adjust to continuous warming by acclimation of their physiological responses (for example, through their rates of photosynthesis and autotrophic respiration) [13] , [14] , [15] . These issues all lead to the question of how and where has the impact of temperature on vegetation productivity changed over the last three decades? Here, with simultaneous use of geographically complete satellite-derived NDVI data, concurrent climate observations and gridded land surface models (see Methods), we show that the strength (correlation) of the linkage between vegetation productivity and temperature has declined from the early 1980s to 2011 for the NH. This weakening relationship is mainly found in temperate and arctic biomes, with possible different causes. Satellite observation We first detrend all quantities to allow focused analysis on correlations in interannual variability. For the entire period of 1982–2011 ( Fig. 1a,b ), the interannual variation of the April to October growing season (GS) NDVI (NDVI GS ) north of 30°N is significantly correlated with the corresponding GS temperature (GT) ( R =0.45, P =0.01), but not with GS precipitation (GP) ( R =−0.009, P =0.96). This is consistent with earlier studies [1] , [3] . However, we found that the yearly correlation coefficient between NDVI GS and temperature significantly declined from 0.72 ( P <0.01) of the first half period (1982–1996) to just 0.32 ( P >0.10) of the second half period (1997–2011) ( Fig. 1c ). To determine whether this decreasing strength of the relationship between NDVI GS and temperature variation is due to a direct temperature physiological response of vegetation, rather than forced through the emergence of controlling effects of other climatic variables, we analyse the change in partial correlation coefficient between NDVI GS and temperature ( R NDVI-GT ). Partial correlation removes statistically the effects of other controlling climate variables, including, for instance, precipitation and cloud cover (see Methods). Here, R NDVI-GT is calculated with a 15-year moving window, still for variables detrended, and results are presented in Fig. 1d . This shows that R NDVI-GT also decreased and with a high significance level ( P <0.01) from 1982 to 2011. Further, this decline of R NDVI-GT is robust to different GS definitions (May–September, May–October, or to the definition of the GS as the period with greenness level >25% or 50% of the amplitude of the seasonal cycle of NDVI for each year, Fig. 1d ). Similar results are also observed when all variables are not detrended ( Supplementary Fig. 1a ), annual precipitation from previous November to current October is used instead of GS precipitation only ( Supplementary Fig. 1b ), or satellite-observed leaf area index [16] is used instead of NDVI as a proxy of vegetation productivity ( Supplementary Fig. 1c ). These results point out to a recent decreasing strength of the direct vegetation response to temperature variation in NH over the last three decades at the continental scale. The loss of a significant correlation between NDVI GS and temperature in the recent period 1997–2011 hinders calculation of changes in the temperature sensitivity of NDVI GS (regression slope), as this sensitivity can no longer be statistically defined. 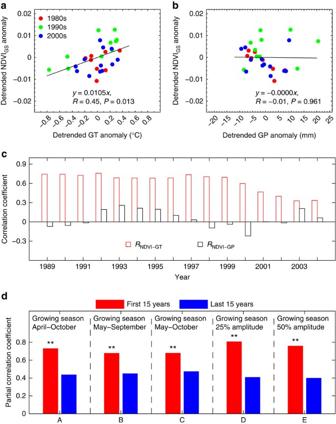Figure 1: The linkage between spatially averaged GS NDVI and climate. Relationship of detrended anomalies of NDVIGSwith (a) GS temperature (GT) and (b) GS precipitation (GP) for the whole study period of 1982–2011. The lines inaandbrepresent the linear regressions of NDVIGSversus GT (a) and GP (b). (c) Changes in the correlation coefficient between NDVIGSand GT, and between NDVIGSand GP after applying 15-year moving windows (all variables detrended for each corresponding window). Thexaxis is the central year of the 15-year moving window (for example, 1990 stands for a moving window from 1983 to 1997). Fora,bandc, GS is defined as April–October. (d) The partial correlation coefficient of NDVIGSand GT (RNDVI-GT) for the first 15 years and the last 15 years with 5 different definition of GS. GS is defined as April–October, May–September, May–October, months with NDVI exceeding 25% of its seasonal amplitude and months with NDVI exceeding 50% of its amplitude, respectively. **Significant correlation atP<0.05. Figure 1: The linkage between spatially averaged GS NDVI and climate. Relationship of detrended anomalies of NDVI GS with ( a ) GS temperature (GT) and ( b ) GS precipitation (GP) for the whole study period of 1982–2011. The lines in a and b represent the linear regressions of NDVI GS versus GT ( a ) and GP ( b ). ( c ) Changes in the correlation coefficient between NDVI GS and GT, and between NDVI GS and GP after applying 15-year moving windows (all variables detrended for each corresponding window). The x axis is the central year of the 15-year moving window (for example, 1990 stands for a moving window from 1983 to 1997). For a , b and c , GS is defined as April–October. ( d ) The partial correlation coefficient of NDVI GS and GT ( R NDVI-GT ) for the first 15 years and the last 15 years with 5 different definition of GS. GS is defined as April–October, May–September, May–October, months with NDVI exceeding 25% of its seasonal amplitude and months with NDVI exceeding 50% of its amplitude, respectively. **Significant correlation at P <0.05. Full size image We analysed the trend of R NDVI-GT separately for 30°N–60°N and above 60°N, and found a significant decrease in R NDVI-GT in both latitude bands ( Supplementary Figs 2 and 3 ). The change of R NDVI-GT is spatially heterogeneous and the declining trend of R NDVI-GT is mostly observed in the temperate and the arctic regions ( Fig. 2a ). Analysing partial correlations over the temperate band south of 50 o N excluding Tibet and subtropical forests, NDVI GS is negatively correlated with GT ( Fig. 2a ), but is also positively correlated with GP ( Supplementary Figs 4 and 5 ), indicating a co-effect of water limitation on interannual NDVI variability. This is consistent with the hypothesis that plant productivity in temperate ecosystems is subject to soil moisture limitation during summer [5] , [17] , [18] . Further, we find that much of the temperate region is experiencing an enhancement of its negative R NDVI-GT ( Fig. 2a ). In contrast to temperate regions, NDVI GS is positively correlated with temperature above that of 50°N, but the partial correlations R NDVI-GT trends are different between Eurasia and North America ( Fig. 2a ). Eurasia boreal regions show more areas with decreasing R NDVI-GT than that of North America, where R NDVI-GT trends are of opposite sign between northern and southern areas (roughly across the 60°N latitude boundary; Fig. 2a ). North of this boundary, R NDVI-GT decreased with time, but R NDVI-GT continued to increase in the south, notably in the southern part of Hudson Bay ( Fig. 2a and Supplementary Fig. 5 ). 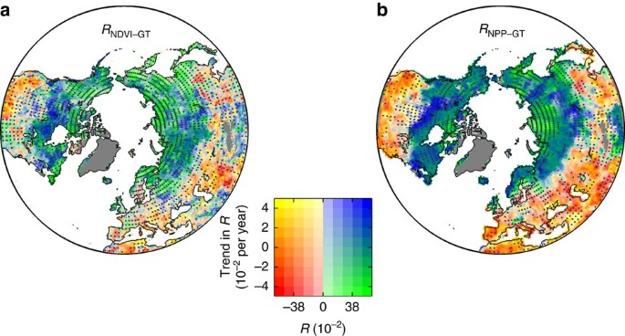Figure 2: Spatial distribution of the partial correlation coefficient of vegetation productivity and climate. (a) Partial correlation coefficient (RNDVI-GT) between GS NDVI (NDVIGS) and GS temperature (GT); (b) partial correlation coefficient (RNPP-GT) between ten models estimated average of GS net primary productivity (NPPGS) and GT. GS is defined as April–October. The horizontal axis of the colour legend is calculated for the entire study period, andR= ±0.38 corresponds to the 0.05 significance levels for the entire study period. Fifteen-year moving windows are used to estimate the trend ofR(the vertical axis of the colour legend). All variables are detrended for the corresponding period. To calculated its partial correlation versus GT, GS precipitation and cloud cover are controlled for. Yellow and red colour indicates a negative correlation of NDVIGS(or NPPGS) and GT, while yellow colour stands for an increasing trend in the correlation and red stands for a decreasing trend. Blue and green colour indicates a positive correlation of NDVIGS(or NPPGS) and GT, while blue colour stands for an increasing trend and green stands for a decreasing one. The dots indicates the regions with significant trend inRNDVI-GT(orRNPP-GT) (P<0.05). Figure 2: Spatial distribution of the partial correlation coefficient of vegetation productivity and climate. ( a ) Partial correlation coefficient ( R NDVI-GT ) between GS NDVI (NDVI GS ) and GS temperature (GT); ( b ) partial correlation coefficient ( R NPP-GT ) between ten models estimated average of GS net primary productivity (NPP GS ) and GT. GS is defined as April–October. The horizontal axis of the colour legend is calculated for the entire study period, and R = ±0.38 corresponds to the 0.05 significance levels for the entire study period. Fifteen-year moving windows are used to estimate the trend of R (the vertical axis of the colour legend). All variables are detrended for the corresponding period. To calculated its partial correlation versus GT, GS precipitation and cloud cover are controlled for. Yellow and red colour indicates a negative correlation of NDVI GS (or NPP GS ) and GT, while yellow colour stands for an increasing trend in the correlation and red stands for a decreasing trend. Blue and green colour indicates a positive correlation of NDVI GS (or NPP GS ) and GT, while blue colour stands for an increasing trend and green stands for a decreasing one. The dots indicates the regions with significant trend in R NDVI-GT (or R NPP-GT ) ( P <0.05). Full size image For the boreal and arctic band, there is a nonsignificant correlation between NDVI and GP (see slightly negative R NDVI-GP values in Supplementary Fig. 4a ). This weak negative value of R NDVI-GP may be attributed to the coincident reduction of incoming solar radiation [19] , [20] during wet years ( Supplementary Fig. 6 ). To investigate the effect of solar radiation on vegetation productivity, we investigated partial correlations of NDVI with shortwave radiation interannual fluctuations ( R NDVI-SR , Supplementary Fig. 7 ). In general, these correlations with radiation are weaker than those found for temperature and precipitation ( Fig. 2a and Supplementary Fig. 4a ). They also vary in sign, suggesting that a positive solar radiation anomaly could either increase the photosynthetic response reflected by a positive NDVI anomaly, or in some instances cause soil moisture depletion from increased transpiration with the opposite effect. The positive value of R NDVI-SR in the high latitude regions thus suggests that vegetation productivity of these regions is not only limited by temperature, but also by solar radiation [5] . Process-based model simulations To gain additional insights on the drivers of the changes in R NDVI-GT , we analyse the response of vegetation productivity to climate variables using the output from ten different global vegetation models (TRENDY ensemble, see Methods). Outputs from these models forced by observed climate fields and changing CO 2 concentration are analysed for their predictions during the period 1982–2010 (see Methods). Net primary productivity (NPP) is chosen as a model diagnostic representative of observed GS-integrated NDVI (similar results are also found for gross primary productivity (GPP), Supplementary Fig. 8a,b ). After detrending all data, we find that modelled NPP and GPP are both significantly positively ( P <0.05) correlated with observed NDVI over 47% of the NH. Despite their different structure, the ten models produce similar spatial patterns of the partial correlation coefficients between NPP and temperature interannual variations ( R NPP-GT ) ( Supplementary Fig. 9 ). Comparing Fig. 2a with Fig. 2b shows that the spatial patterns of modelled R NPP-GT are comparable to the satellite data analysis. The models faithfully simulate positive average values of R NPP-GT in high-latitude regions and negative values in temperate regions, similar to that for R NDVI-GT . For precipitation, however, the responses of modelled NPP are different from that of NDVI. For example, unlike R NDVI-GP , a positive correlation between NPP and precipitation ( R NPP-GP ) is generally modelled in the high-latitude regions. The area with significant positive R NPP-GP , when estimated by the models, is about twice that diagnosed from satellite observations (6%) ( Supplementary Figs 10 and 11 ). Such an overestimation of the positive sensitivity of vegetation productivity to precipitation change by models has been noted in recent studies [18] , [19] . Now looking at trends over the last 30 years, the geographic patterns of the R NPP-GT trend is broadly similar to that of R NDVI-GT trend ( Fig. 2 ), providing two lines of evidence (that is, both Earth Observing and model-based) for changes in the interannual response of vegetation productivity to temperature, against a background of climate change. Yet, when aggregated at the continental scale, most models generally do not show significant negative trend of R NPP-GT (except for Sheffield–DGVM and VEGAS, Supplementary Fig. 12 ). This is because models produce a smaller area with decreasing trend of R NPP-GT ( Fig. 2 and Supplementary Fig. 11 ) than the NDVI observations. Mechanisms Mechanisms causing the observed decline in R NDVI-GT cannot be elucidated from statistical analysis alone. We focus here on two possible mechanisms: the effect of drought trends attenuating the response of NDVI to temperature variability and the effect of increasing occurrence of extreme hot days during the 2000s despite stalled mean temperature in the NH [21] . Drought has increased in temperate regions during the last decades [9] , particularly in the central and western United States, northeast China and Central Asia ( Supplementary Figs 13 and 14 ). Drought reduces water availability for plant growth during the GS and extreme drought can even cause hydraulic failure, therefore offsetting or masking positive R NDVI-GT values. In addition, extreme hot days (T × 90p, the number of days with temperature higher than the 90th percentile of the GS temperature distribution during 1982–2011) show a positive trend ( Supplementary Fig. 15 ). The increased occurrence of hot extremes can reach above the range of temperate and boreal vegetation acclimation conditions and attenuate the sensitivity of productivity to temperature [22] ; for instance, by increasing the fraction of assimilates needed for maintenance, leading to reduced R NDVI-GT . To gain insights about these two mechanisms, we show in Fig. 3 the trends of R NDVI-GT within phase space of changes in precipitation and trend in T × 90p for the temperate and boreal (30–60°N) and for the northern boreal and arctic latitude bands (above 60°N). 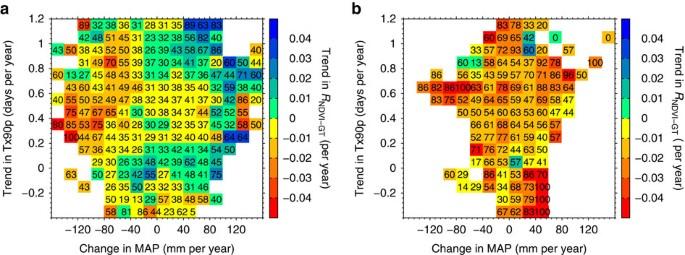Figure 3: Average trend ofRNDVI-GTin a climate phrase space. Here,RNDVI-GTis the partial correlation coefficient between GS NDVI (NDVIGS) and GS temperature (GT) shown inFig. 2a, and the climate space is delineated by changes in GS hot extreme days and mean annual precipitation (MAP). The number in each climate space indicates the percentage (%) of pixels with significant trend inRNDVI-GTfor each climate space (if the average of trend inRNDVI-GTis positive, then the percentage of pixels with significant and positive of trend inRNDVI-GTwas shown; otherwise, the percentage of pixels with significant and negative of trend inRNDVI-GTwas shown). The hot extreme days are defined as the 90th percentile warm day frequency (T × 90p), that is, the number of days above the 90th percentile21. The change in MAP is calculated as the difference between the mean of 1997–2011 and the mean of 1982–1996. The trend ofRNDVI-GTis presented separately for regions over (a) 30°N–60°N and (b) 60°N–90°N. Figure 3: Average trend of R NDVI-GT in a climate phrase space. Here, R NDVI-GT is the partial correlation coefficient between GS NDVI (NDVI GS ) and GS temperature (GT) shown in Fig. 2a , and the climate space is delineated by changes in GS hot extreme days and mean annual precipitation (MAP). The number in each climate space indicates the percentage (%) of pixels with significant trend in R NDVI-GT for each climate space (if the average of trend in R NDVI-GT is positive, then the percentage of pixels with significant and positive of trend in R NDVI-GT was shown; otherwise, the percentage of pixels with significant and negative of trend in R NDVI-GT was shown). The hot extreme days are defined as the 90th percentile warm day frequency (T × 90p), that is, the number of days above the 90th percentile [21] . The change in MAP is calculated as the difference between the mean of 1997–2011 and the mean of 1982–1996. The trend of R NDVI-GT is presented separately for regions over ( a ) 30°N–60°N and ( b ) 60°N–90°N. Full size image We find that in the band 30–60°N, the trend of R NDVI-GT is more often negative in regions that have experienced a reduction in precipitation (increased drought) between the first and the last parts of the past 30 years ( Fig. 3a ). However, there is no significant change in the trend of R NDVI-GT along the gradient of increasing number of hot days ( Fig. 3a ). This result suggests that for northern temperate vegetation, where water is a limiting factor for vegetation growth, lower precipitation rather than increased hot days is associated with the decline of R NDVI-GT . Decrease in precipitation can reduce soil water content and indeed we find that a stronger negative R NDVI-GT or R NPP-GT usually occurs ( Fig. 2 ) in areas with decreasing soil moisture from models ( Supplementary Fig. 14 ). In contrast, NDVI observations and most models show an upward trend of R NDVI-GT and R NPP-GT in the lower Hudson Bay ( Fig. 2 and Supplementary Fig. 9 ), where models produce increasing soil moisture ( Supplementary Fig. 14 ). This is also supported by the spatial correlation analyses between local partial correlation coefficient ( R NDVI-GT ) and precipitation for 5° by 5° moving windows. This positive spatial correlation between R NDVI-GT and precipitation indicates that a stronger (and positive) association of vegetation productivity to temperature occurred in areas receiving more precipitation ( Supplementary Fig. 16 ). By contrast, in the Northern boreal and Arctic areas (above 60°N) a decline of R NDVI-GT is observed across most regions, regardless of their precipitation trend ( Fig. 3b ). Thus, the weakening R NDVI-GT in the arctic regions is unlikely caused by changes in precipitation. On the other hand, the number of hot days has also increased in most arctic regions over the past 30 years ( Supplementary Fig. 15 ), which could reduce R NDVI-GT , because the sensitivity of vegetation growth to heat waves is generally different from that to normal temperature. Yet, the trend in R NDVI-GT does not show a strong tendency along the gradient of the trend of hot extreme days ( Fig. 3b ), suggesting that other mechanisms may also be responsible for the reduced R NDVI-GT in the arctic region. For example, the decreasing trends of R NDVI-GT when climate becomes warmer can be qualitatively explained if the physiological response of photosynthesis to temperature follows a nonlinear (convex) curve with lower sensitivity under warmer conditions [23] , [24] . Such a response to temperature is expected to weaken the correlation strength between vegetation growth and temperature in warmer years. To test this mechanism, we compare R NDVI-GT and its change between cold and warm years north of 60°N in Fig. 4 . The data in this figure indicate that R NDVI-GT for cold years is systematically higher than for warm years. Moreover, there is a more significant and accelerating decrease of R NDVI-GT for warm years as compared with that of cold years ( Fig. 4 ), implying a decoupling or even a reverse correlation between NDVI and temperature with continuous climate warming. In addition, woody encroachment and increase of the contribution of shrubs to total productivity into tundra areas under climate warming may also potentially contribute to the observed decrease in R NDVI-GT due to the very different responses of grassland and woody vegetation to temperature change [25] , [26] , [27] . For instance, shrubs were shown to have a positive response to temperature only in July, whereas grasses respond to GT [27] . 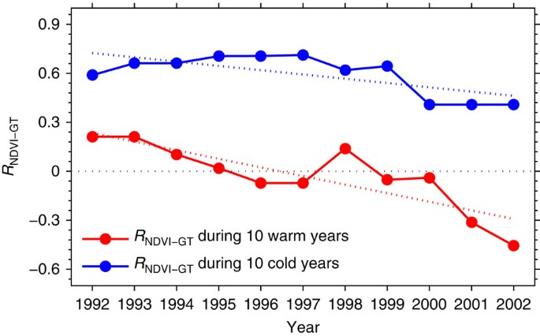Figure 4: Changes inRNDVI-GTover the Arctic in warm and cold years. Here,RNDVI-GTis the partial correlation coefficient between GS NDVI (NDVIGS) and GS temperature (GT). Year on the horizontal axis is the central year of each 20-year moving window used to deriveRNDVI-GT(for example, 1992 represents period 1982–2001 in the 20-year time window). For each 20-year series, we divide the 20 years into two groups based on their ranks in GS temperature: the 10 years with higher GS temperature are defined as warm years, and the other 10 years are cold years. We then calculateRNDVI-GTfor warm and cold years, separately, through controlling for corresponding GS precipitation and cloud cover. Over the past three decades,RNDVI-GTshows a significant decreasing trend for both warm (R2=0.71,P=0.001) and cold (R2=0.49,P=0.016) years; andRNDVI-GTfor cold years is higher than that of warm years over all the 20-year series. Figure 4: Changes in R NDVI-GT over the Arctic in warm and cold years. Here, R NDVI-GT is the partial correlation coefficient between GS NDVI (NDVI GS ) and GS temperature (GT). Year on the horizontal axis is the central year of each 20-year moving window used to derive R NDVI-GT (for example, 1992 represents period 1982–2001 in the 20-year time window). For each 20-year series, we divide the 20 years into two groups based on their ranks in GS temperature: the 10 years with higher GS temperature are defined as warm years, and the other 10 years are cold years. We then calculate R NDVI-GT for warm and cold years, separately, through controlling for corresponding GS precipitation and cloud cover. Over the past three decades, R NDVI-GT shows a significant decreasing trend for both warm ( R 2 =0.71, P =0.001) and cold ( R 2 =0.49, P =0.016) years; and R NDVI-GT for cold years is higher than that of warm years over all the 20-year series. Full size image Rising CO 2 also has the effect to reduce transpiration and increase water use efficiency, as well as to increase productivity in the absence of nutrient limitation. We used additional model output to investigate NPP–climate relationships when removing the simulated response of NPP to increasing CO 2 (+50 p.p.m.) that occurred in parallel to climate change over the period of analysis. When removing the effects of increasing CO 2 on the modelled NPP–climate relationship analysis, the resulting R NPP-GT partial correlations ( Supplementary Fig. 17 ) are found to be almost identical to those obtained when both climate and CO 2 vary ( Fig. 2 ). Hence, at least in models, the correlation changes observed do not depend on the effect of rising CO 2 fertilization, but we note that only one model included elevated CO 2 and nitrogen interactions. Further research is needed, combining process studies (for example, ecosystem warming experiments) with large-scale data to further understand the mechanisms that underlay the observed decline in the correlation between temperature and vegetation growth in each region. Multiple uncertainties remain in understanding the evolution of NH vegetation. These may include processes not modelled, incorrect model drivers of radiation and extreme events, or ill-parameterized descriptions of the vegetation response to a changing hydrological cycle, for example, the effect of snow change on vegetation productivity [28] . Resolving some of these may aid to resolve the overestimation of precipitation sensitivity of vegetation productivity by models in comparison with the satellite-based data. Other indirect climate effects such as insects [29] , frost damage during spring, fire disturbances [8] , exposure to high surface ozone concentration, background nutrient limitations and changes in nutrient availability [30] , land use and land management changes (for example, over-grazing by reindeers in the Taymyr Peninsula region where a strong decrease of R NDVI-GT is observed [31] ) also have the potential to attenuate the observed NDVI–climate interannual correlations. These factors could also explain some of the differences in the spatial patterns of observed versus modelled NDVI–climate correlations (that is, Fig. 2a versus Fig. 2b ), as many of these processes are not systematically included in terrestrial ecosystem models. However, despite large uncertainties, satellite NDVI measurements and multi-model estimates of NPP and GPP provide evidence of an overall decrease in the interannual correlation between temperature and productivity over the last three decades. Because of the relatively short time period of satellite data, we cannot say whether these observed changes reflect decadal variability, or a long-term transition in the vegetation–climate relationship. NPP from TRENDY models show that there is decadal variability in R NPP-T over the last century ( Supplementary Fig. 18 ), but we also note that these TRENDY models did not capture the observed change of R NDVI-GT during the last three decades at NH scale. Analysis of longer time series of proxies, such as tree ring growth index [32] , should provide further insights on this question. We also found compelling indications that change in soil moisture is an important process that modulates the temperature–productivity correlations, although the models used in this study may be presently less trusted to fully describe this. It is not straightforward to link changes in NDVI–temperature relationships with changes in the net carbon balance of northern ecosystems that has an impact on seasonal [33] and spatial gradients of atmospheric CO 2 , because of the concurrent response of respiration and disturbances to temperature. Further study focusing on both the temperature dependence of vegetation productivity and ecosystem respiration and their temporal trajectory is needed. Data sets Investigating satellite-derived vegetation greenness and its association with climate provides useful information for the complex coupling of biosphere and atmosphere. The biweekly NDVI data of 1982–2011 used in this study were obtained from the GIMMS (Global Inventory Modeling and Mapping Studies) team, with a spatial resolution of 0.083°. They were further aggregated to 0.5° × 0.5° to match the resolution of meteorological data. The calibrated Advanced Very High Resolution Radiometer (AVHRR)-NDVI data have been successfully used in many studies of vegetation monitoring [34] , [35] , although the original AVHRR sensor series were not designed for vegetation monitoring and thus suffered from lack of onboard calibration and navigation/georeferencing problems. Here we used the third-generation GIMMS-NDVI3g data, which have been corrected for sensor degradation, intersensor differences, cloud cover, solar zenith angle, viewing angle effects due to satellite drift and volcanic aerosols [36] , [37] . Monthly climatology (including air temperature, precipitation and cloud cover) data with spatial resolution of 0.5° × 0.5° were compiled from meteorological data stored at the Climate Research Unit, University of East Anglia (CRU TS 3.2) [38] . The 2.5° × 2.5°gridded data of monthly PDSI calculated from a simple water balance model [9] were provided by the University Corporation for Atmospheric Research. Similar to the PDSI_PM used in Sheffield et al. [39] , evaporation in this PDSI data set was also calculated using a more sophistical Penman–Monteith equation. Ecosystem models In this study, we simulated annual NPP and soil moisture using ten process-based ecosystem models: HyLand, Lund-Potsdam-Jena DGVM (LPJ), ORCHIDEE, Sheffield–DGVM, JULES, LPJ_GUESS, CLM4C, CLM4CN, OCN and VEGAS. All models followed the protocol described by the historical climate carbon cycle model intercomparison project (Trendy) ( http://dgvm.ceh.ac.uk/system/files/Trendy_protocol%20_Nov2011_0.pdf ) [40] , [41] . All models used prescribed static vegetation maps. Each model was run from its pre-industrial equilibrium (assumed at the beginning of the 1900s) to 2010 with two scenarios: in S1 scenario models are forced only by historical change of atmospheric CO 2 concentrations, and in S2 scenario models are forced by both observed historic climate changes and rising CO 2 concentrations. All models can estimate NPP; six of ten models provide leaf area index and seven of ten models provide soil moisture information. Analysis This study covered the vegetated areas (defined as area with mean GS NDVI during 1982–2011 larger than 0.05) north of 30°N and the study period was 1982–2011 based on the availability of satellite observations and meteorological data sets. GS was defined as April–October, but results from other GS definitions such as May–September and May–October were also presented in Supplementary Figures 1–18 , for robustness test. Change in GS length for each year was also taken into account through defining GS as the period with greenness level >25% or 50% of the amplitude of the seasonal cycle of NDVI. The temperature variation signal in NDVI was calculated as the partial correlation coefficient between GS NDVI and GS temperature ( R NDVI-GT ) after statistically controlling for interannual variation in precipitation and cloud cover over a 15-year moving window. Hence, R NDVI-GT can be influenced by general background climate changes, occurring over periods of 15 years or longer. Within each 15-year window, the linear trend derived from the least squares method was removed for both NDVI GS and climate time series. Using similar method, we also calculate the temperature variation signal in NPP estimated from the carbon cycle models. All these analyses were first performed for the entire NH (>30°N) and then for each pixel. An alternative method to extract the climate variation signal in NPP is to use two scenarios of model simulations ( http://dgvm.ceh.ac.uk/system/files/Trendy_protocol%20_Nov2011_0.pdf ). In S1 scenario, models are driven by historical change of atmospheric CO 2 concentration; in S2 scenario, models are driven by historical change of both atmospheric CO 2 concentration and climate. The difference of simulated NPP in these two scenarios should represent the climate impacts on vegetation productivity. We also analysed simulated NPP with this approach, resulting in similar conclusions ( Supplementary Fig. 17 ). How to cite this article: Piao, S. et al. Evidence for a weakening relationship between interannual temperature variability and northern vegetation activity. Nat. Commun. 5:5018 doi: 10.1038/ncomms6018 (2014).